Diverse manifestations of the mid-Pleistocene climate transition The mid-Pleistocene transition (MPT) is widely recognized as a shift in paleoclimatic periodicity from 41- to 100-kyr cycles, which largely reflects integrated changes in global ice volume, sea level, and ocean temperature from the marine realm. However, much less is known about monsoon-induced terrestrial vegetation change across the MPT. Here, on the basis of a 1.7-million-year δ 13 C record of loess carbonates from the Chinese Loess Plateau, we document a unique MPT reflecting terrestrial vegetation changes from a dominant 23-kyr periodicity before 1.2 Ma to combined 100, 41, and 23-kyr cycles after 0.7 Ma, very different from the conventional MPT characteristics. Model simulations further reveal that the MPT transition likely reflects decreased sensitivity of monsoonal hydroclimate to insolation forcing as the Northern Hemisphere became increasingly glaciated through the MPT. Our proxy-model comparison suggests varied responses of temperature and precipitation to astronomical forcing under different ice/CO 2 boundary conditions, which greatly improves our understanding of monsoon variability and dynamics from the natural past to the anthropogenic future. The Pleistocene climate is characterized by significant glacial–interglacial changes in high-latitude ice volume [1] , [2] , [3] , global ocean temperature [4] , sea level [5] , and monsoonal climate [6] . All these variables inherently interacted to generate a remarkable transition of the ice-age cycles from 41-kyr to 100-kyr cycles between 1.2 and 0.7 Ma, called the mid-Pleistocene transition (MPT) [2] , [7] , [8] . The MPT might be triggered by a nonlinear response to astronomical forcing [9] induced by a secular CO 2 decrease and/or progressive regolith erosion [10] , [11] , [12] . This transition is particularly apparent in numerous proxy indicators that are sensitive to changing glacial boundary conditions [3] , [4] , [5] , [6] , [11] , [13] . At middle and low latitudes, however, the proxies of monsoon-induced wind and hydroclimate changes in the Arabian Sea and East Asia display prominent precession cycles during the middle-to-late Pleistocene [14] , [15] . Simulations with different climate models show that global monsoon changes are sensitive to changes in insolation, CO 2 concentration, and ice volume [16] , [17] , [18] , [19] . Synthesis of Chinese loess, paleolake, and speleothem records confirms that the Asian summer monsoon variation was induced by combined effects of astronomical, ice, and CO 2 forcing [20] . However, the relative roles of the insolation and coupled ice/CO 2 changes in driving orbital-scale monsoon variability remain controversial due to the spatial divergence and complexity of the proxy sensitivity to precipitation and temperature changes [14] , [15] , [19] , [20] , [21] , [22] . Here we present a centennial-resolution δ 13 C record of inorganic carbonate (δ 13 C IC ) of a thick loess sequence from the northwestern Chinese Loess Plateau (CLP), a region sensitive to orbital-to-millennial-scale monsoon variability [22] , [23] . Magnetostratigraphy and pedostratigrahpy, together with burial dating, provide a reliable chronology of the loess–paleosol sequences accumulated over the past ~1.7 Ma. Loess δ 13 C IC , a sensitive monsoon proxy, offers novel insights into Pleistocene monsoon variability and dynamics. Unlike the conventional expression of the MPT, our results reveal a compelling transition of the dominant rhythm in coupled monsoon–vegetation system from 23-kyr to combined 23-, 41-, and 100-kyr cycles across the MPT. Setting and sampling CLP climate is characterized by seasonal changes in temperature and precipitation. Summer is the warm and humid season due to the influence of the summer monsoon, which transports heat and water vapor from the low-latitude oceans. The summer precipitation from May to September contributes to the annual precipitation by 60–75% and results in strong pedogenesis of the loess–paleosol sequences. In contrast, winter is the cold and dry season associated with strong winter monsoon wind, which is linked to the Siberian–Mongolian high-pressure system. The winter monsoon transports vast of dust particles from inland Asia to the downwind CLP. Therefore, Chinese loess, as a unique continental archive, can document multi-scale monsoon variability linked to past climate changes in both high- and low-latitude regions [20] , [21] , [22] , [23] , [24] , [25] , [26] . The Jingyuan loess sequence (JY, 36.35°N, 104.6°E, 2,210 m above sea level) is located at the depositional center of modern dust storms on the northwestern CLP (Fig. 1 ). A 430-m core was retrieved from the highest terrace of the Yellow River near Jingyuan County. The JY core consists of a 427-m loess deposit underlain by a 3-m gravel layer. A 40-m outcrop was excavated nearby to collect parallel samples spanning the last interglacial–glacial cycle. Continuous U-channel and discrete cube samples were taken from the split cores for alternating-field and thermal demagnetization measurements, respectively (Methods). Three quartz samples were chosen from the underlying gravel layer for 26 Al/ 10 Be burial dating (Supplementary Fig. 1 ). Powder samples were taken at 10-cm intervals for magnetic susceptibility, grain size, and δ 13 C IC analyses. Fig. 1 Location of JY loess core and representative loess profiles on the Chinese Loess Plateau (CLP). Black dots denote four classic loess profiles, which have been investigated intensively as the Quaternary stratotype sections [25] , [26] , [27] , [28] , [29] , [30] , [31] . Red dot indicates the Jingyuan loess profile accumulated on the ninth terrace of the Yellow River in the northwestern CLP [23] , [41] Full size image Magnetostratigrahy and pedostratigrahy Magnetic measurements and demagnetization spectra indicate that the JY loess sediments contain dominantly coarse-grained domain magnetite, which records the primary detrital remanent magnetization (Supplementary Figs. 2 and 3 ). Paleomagnetic results reveal that the Brunhes/Matuyama (B/M) boundary is recorded at the S 7 /L 8 boundary and the Jaramillo subchron is located within S 10 –L 13 (Fig. 2 ). The magnetostratigraphy of the JY loess sequence is well correlated with that of classic loess profiles from the central CLP [27] , [28] , [29] , [30] , [31] , e.g., the B/M boundary at the top L 8 and the Jaramillo subchron between S 10 and L 13 (Supplementary Fig. 4 ). Correlation of the JY magnetostratigrapy with geomagnetic polarity timescale [32] indicates that the Olduvai subchron is not recorded at the JY section (Fig. 2 ). Fig. 2 Polarity and proxy variations of the JY loess sequence. a Geomagnetic polarity timescale (GPTS) [32] , [33] . b Magnetic susceptibility (MS) and magnetostratigraphy of Luochuan (LC) profile [27] , [31] . c JY δ 13 C IC , mean, and magnetostratigrahy. The magnetostratigraphy is derived from inclination results measured by the alternating-field (AFD, light blue) and thermal (THD, purple) demagnetization methods. Dashed lines indicate the positions of paleomagnetic reversals (B/M Brunhes/Matuyama boundary, J Jaramillo, O Olduvai). Orange bars denote thick loess marker layers Full size image In addition, several normal excursions are evident in the inclination results below the B/M boundary, which either resulted from remagnetization of coarse-grained magnetic particles or are related to genuine geomagnetic excursions [33] , [34] . Previous studies have deliberately evaluated the fidelity of these relatively short-lived directional anomalies, which could indicate remagnetization caused by physical realignment of magnetic grains in wetter conditions [35] or by viscous remanent magnetization overprinting on the coarse-grained eolian magnetic particles [36] . The general correspondences between these short-lived directional anomalies and the grain-size curve seems supporting the remagnetization mechanism. Loess–paleosol alternations can be reliably recognized and correlated throughout the entire CLP using magnetic susceptibility and grain-size variations. While the pedogenesis inferred from the magnetic susceptibility is relatively weak at the JY loess sequence, mean grain-size and δ 13 C IC variations faithfully document the loess–paleosol alternations from S 23 to S 0 (Fig. 2 ), consistent with the pedostratigraphy of other typical Chinese loess profiles [25] , [26] , [27] , [28] , [29] , [30] , [31] (Supplementary Fig. 4 ). Seven thick loess units (L 1 , L 2 , L 5 , L 6 , L 9 , L 15 , and L 23 ) can be readily identified as marker layers for pedostratigrapic correlation. In between these marker layers, JY loess–paleosol alternations from S 23 to S 0 can be easily counted from the mean grain-size variations, which are quite similar to large-amplitude grain-size fluctuations of other representative loess profiles (Supplementary Fig. 4 ). 26 Al/ 10 Be burial dating The concentrations of 26 Al and 10 Be in quartz were derived from the measured isotopic ratios (Methods). 10 Be value was adjusted to match the currently accepted value [37] , and the 26 Al/ 27 Al ratio was normalized to standards [38] . For the Jingyuan location (latitude 36.35°N and elevation 2210 m) [39] , cosmogenic nuclide production rates were estimated to be 150.42 and 22.09 atoms per gram per year for 26 Al and 10 Be, respectively. Burial ages were calculated by iteratively solving equations without considering the post-burial cosmogenic nuclide production [40] . 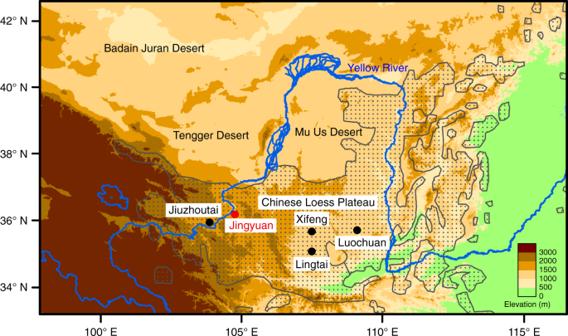Fig. 1 Location of JY loess core and representative loess profiles on the Chinese Loess Plateau (CLP). Black dots denote four classic loess profiles, which have been investigated intensively as the Quaternary stratotype sections25,26,27,28,29,30,31. Red dot indicates the Jingyuan loess profile accumulated on the ninth terrace of the Yellow River in the northwestern CLP23,41 Burial ages of three samples from the same gravel layer vary from 1.62 to 1.87 Ma, with uncertainties of 0.14–0.47 Ma (Table 1 ). The average age of basal gravel layer was estimated to be 1.73 ± 0.13 Ma, which is consistent with the timing of Lanzhou loess sequence on the ninth terrace of the Yellow River [41] . Integrating the paleomagnetic results and the burial dates suggests that the JY loess sequence accumulated after 1.77 Ma. Table 1 Cosmogenic nuclide concentrations and burial age Full size table Chronology The loess chronology has been generated using both orbital tuning [25] , [26] and a grain-size model [24] , [42] , [43] . These approaches result in almost identical ages of the loess/paleosol boundaries from S 8 to S 0 , matching well with the timing of the glacial/interglacial transitions of benthic δ 18 O stack [3] . During early-to-middle Pleistocene, orbital tuning can provide better constraints on the timing of the loess/paleosol boundaries compared to the grain-size age model approach due to the capacity for more time control points [25] , [26] . However, orbital tuning can involve obliquity and precession imprints in the age model and thus hamper our assessment of the periodicity changes across the MPT. Owing to the strong similarity of loess–paleosol alternations between the Jingyuan core and other classic loess profiles, a pedostratigraphic age model can be developed using only 12 tie points to match 7 thick loess layers to the stacked grain-size time series [25] , [26] (Fig. 3 ). The age model was refined by interpolation between 12 time controls using the weighted grain-size model [24] . The basal age of the JY loess was estimated to be ~1.73 Ma, and the sedimentation rate varies between 10 and 70 cm/kyr. The age model can be verified by a robust correlation of the Jingyuan grain-size variation with stacked loess grain-size [25] , [26] and benthic δ 18 O records [3] (Fig. 3 ). Fig. 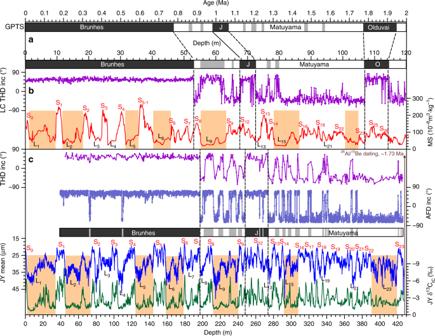Fig. 2 Polarity and proxy variations of the JY loess sequence.aGeomagnetic polarity timescale (GPTS)32,33.bMagnetic susceptibility (MS) and magnetostratigraphy of Luochuan (LC) profile27,31.cJY δ13CIC, mean, and magnetostratigrahy. The magnetostratigraphy is derived from inclination results measured by the alternating-field (AFD, light blue) and thermal (THD, purple) demagnetization methods. Dashed lines indicate the positions of paleomagnetic reversals (B/M Brunhes/Matuyama boundary, J Jaramillo, O Olduvai). Orange bars denote thick loess marker layers 3 Comparison of JY grain-size time series with stacked loess grain-size and benthic δ 18 O. a Benthic δ 18 O stack [3] . b Loess grain-size (GS) stack [25] . c Quartz grain-size (QGS) stack [26] . d JY mean grain-size on age scale. e JY mean grain-size on depth scale. Dashed lines denote that the chronology was generated by matching the timing of seven loess marker layers (L 1 , L 2 , L 5 , L 6 , L 9 , L 15 , and L 23 ) to stacked grain-size time series. Orange and blue bars indicated the correlation of thick marker layers and other loess units to glacial stages Full size image Reliability of this age model can be further assessed from the raw depth spectra over three depth intervals (Fig. 4a ). The cyclicity ratios (27 m/11.5 m = 2.3 and 11.5 m/5.5 m = 2.1) in the depth spectra are consistent with the orbital ratios (100kyr/41kyr = 2.4 and 41kyr/21kyr = 2.0). Notably, a 5.5-m cycle is evident throughout the entire sequence and becomes dominant below L 15 . Applying a 5.5 m = 21kyr relationship results in a pedostratigraphic correlation of the lower portion to L 15 –S 23 and a basal age of ~1.73 Ma. Based on a linear depth–time transformation, an intrinsic cyclicity shift is evident from 23-kyr below L 15 (1.2–1.7 Ma) to 100-kyr above L 9 (0–0.9 Ma) (Fig. 4b ). Fig. 4 Spectral results of JY δ 13 C IC record. a On depth scale, dominant cyclicity changes from 5.5 to 6.7 m/cycle below L 15 to 19.6-27 m/cycle above L 9 . b The dominant cyclicity on age scale is evidently shifted from 23-kyr before 1.2 Ma (below L 15 ) to 100-kyr after 0.9 Ma (above L 9 ) Full size image Alternatively, applying a 5.5 m = 41kyr relationship could result in a pedostratigraphic correlation of the lower portion to L 15 –S 29 and a classic MPT from 41- to 100-kyr cycles (Methods and Supplementary Fig. 5 ). This would require significantly lower sedimentation rate below L 15 (13.5 cm/kyr) relative to that of the upper portion (25 cm/kyr above L 15 ). Such a remarkable change in the sedimentation rate below and above L 15 is inconsistent with linear age-depth relationships of classic loess profiles on the CLP (Supplementary Fig. 6 ). Moreover, the basal age (~2.2 Ma) estimated from the alternative pedostratigraphic correlation is significantly older than independent paleomagnetic and burial dating results. Thus we consider that the alternative pedostratigraphic correlation is sedimentologically implausible. Loess δ 13 C IC implication Proxies related to vegetation change such as carbon isotopes of organic matter and inorganic carbonate in Chinese loess have been employed to assess coupled monsoon–vegetation changes [44] , [45] , [46] , [47] . Both detrital and pedogenic carbonates are present in the Chinese loess deposits [48] , [49] . Carbon isotopes of the detrital carbonates from dust source areas over inland Asia vary between a narrow range of −0.9‰ to 0.7‰ [22] . Thus the carbon isotope of inorganic carbonate (δ 13 C IC ) in Chinese loess is controlled mainly by two factors: carbon isotopes of pedogenic carbonate and the proportion of pedogenic carbonates [22] , [50] . The vegetation in the western CLP is dominated by C3 plants and its carbon isotopes varied by ~2–3‰ due to the biomass changes at glacial–interglacial timescales [44] , [51] , [52] . The carbon isotopic difference between inorganic carbonate and organic matter indicates that secondary carbonates roughly contribute two thirds of the glacial–interglacial δ 13 C IC fluctuations (~7‰), which is also attributed to changing vegetation density [22] , [44] . To determine the climate-vegetation linkage, the δ 13 C IC results of 20 surface soil samples over the CLP were compared with the precipitation and temperature data over 1981–2010 from the China meteorological data center (Supplementary Fig. 7 ). The correlation between the δ 13 C IC results and mean annual/summer precipitation is quite similar, whereas its correlation with the mean annual temperature is much higher than the mean summer temperature. Correlations between the δ 13 C IC of surface soil samples and climate variables reveal that while both mean annual temperature and precipitation can affect vegetation growth, mean annual summer precipitation likely plays a dominant role in the vegetation growth over the northwestern CLP. Since temperature and precipitation are strongly coupled over the CLP (i.e., warm–humid in summer and cold–dry in winter), loess δ 13 C IC can serve as a sensitive indicator of the monsoon-induced vegetation change during the Pleistocene. The δ 13 C IC records display clear precession and millennial oscillations over the last 140 ka (Fig. 5 ), identical to those in Chinese speleothem and Greenland ice-core records [15] , [53] . During marine isotope stage 5 (MIS 5), three negative peaks in the loess δ 13 C IC exhibit a decreasing trend from MIS 5e to MIS 5a, corresponding to changing summer insolation maxima. Our δ 13 C IC records also exhibit stadial–interstadial oscillations. Thirteen Heinrich-like events revealed by the loess 13 C IC records match well with weak summer monsoon intervals in the speleothem δ 18 O and cold stadials in the Greenland ice core. 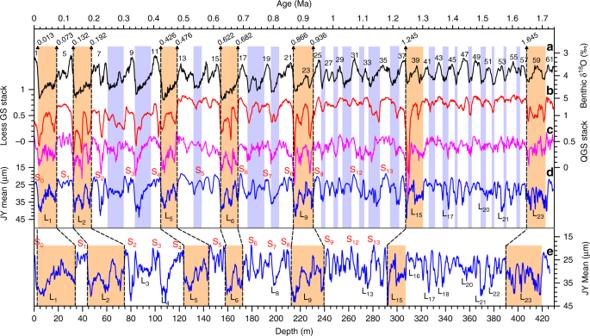Fig. 3 Comparison of JY grain-size time series with stacked loess grain-size and benthic δ18O.aBenthic δ18O stack3.bLoess grain-size (GS) stack25.cQuartz grain-size (QGS) stack26.dJY mean grain-size on age scale.eJY mean grain-size on depth scale. Dashed lines denote that the chronology was generated by matching the timing of seven loess marker layers (L1, L2, L5, L6, L9, L15, and L23) to stacked grain-size time series. Orange and blue bars indicated the correlation of thick marker layers and other loess units to glacial stages High similarity between precession-to-millennial variability in Chinese loess, speleothem, and Greenland ice-core records confirms that our loess δ 13 C IC record is sensitive to both high-latitude temperature and low-latitude hydrological changes. Fig. 5 Proxy variations over the last 140 ka from Greenland ice core, Chinese loess, and speleothem. a Chinese spleothem δ 18 O record [15] . b JY loess δ 13 C IC . c Greenland ice-core δ 18 O record [53] . Dashed lines denote correlations of positive loess δ 13 C IC and speleothem δ 18 O with low Greenland temperature Full size image Sensitivity simulations To estimate the monsoon sensitivity to various forcings, we use the set of 61 experiments with the climate model HadCM3 [54] , which were designed to sample the ensemble of glacial, CO 2 , and astronomical conditions experienced by the land–ocean–atmosphere system during the Pleistocene (Methods). A statistical model (called emulator) is used to interpolate the output of these experiments and to simulate the trajectory of the climate system throughout the Pleistocene. The model results are used to estimate the relative influences of different astronomical parameters (eccentricity, obliquity, and precession) [35] , CO 2 concentrations (180–280 ppmv) [56] , [57] , and discrete levels of glaciation ranging from 1 (Holocene-like) to 11 (Last Glacial Maximum) [54] (Supplementary Fig. 8 ). As the loess δ 13 C IC record is affected by changes in mean annual precipitation (MAP) and temperature (MAT), we focused on these two variables averaged over northern China (30–40°N, 104–120°E), where the precipitation change is more sensitive to summer monsoon intensity [19] . The sensitivity analysis was based on the emulator approach [54] . The emulator is evaluated using a leave-one-out cross-validation approach, which consists of predicting the output of one experiment using the emulator calibrated on all the other experiments. Prediction errors for the MAT and MAP over northern China are well calibrated, and about 2/3 of the prediction errors are within one standard deviation (Supplementary Fig. 9 ). The calibrated emulator is then used for two purposes. First, we estimated the evolution of these indices throughout the Pleistocene to reconstruct the MAP and MAT curves. The MAP and MAT values are the estimated equilibrium response of HadCM3 for forcing conditions spanning the last 1.7 Ma. The climate evolution estimated following this approach considers thus that MAT and MPT are in quasi-equilibrium with the forcing components, including astronomical solutions [55] , ice levels [3] , and CO 2 concentrations [56] , [57] . Next, we estimated the total variances of both MPT and MAT with the emulator, before and after the MPT. The expected variances of these variables caused by the variations of only one or two factors (eccentricity and longitude of perihelion, obliquity, ice, and CO 2 ) were estimated by assuming that the other factors are fixed [54] . Mid-Pleistocene monsoon transition The mean grain-size (an indicator of the winter monsoon intensity [25] , [26] ) and δ 13 C IC (a proxy of monsoon-induced vegetation density [22] , [44] ) records display remarkable changes in both frequency and amplitude around two coarsening loess units (L 15 and L 9 ) (Fig. 2 ). Notably, the δ 13 C IC records show a distinctive transition from rapid oscillations (5.5 and 6.7 m/cycle) below L 15 to low-frequency fluctuations (11.5, 19.6 and 27 m/cycle) above L 9 , representing an intrinsic shift from 23-kyr before 1.2 Ma to 41- and 100-kyr cycles after 0.9 Ma (Fig. 4 ). Over longer timescales, the loess δ 13 C IC record exhibits distinctive glacial–interglacial and precessional variability over the past 1.7 Ma, which differs significantly from both summer insolation and benthic δ 18 O (Fig. 6 ). In the loess δ 13 C IC records, precessional cycles were dominant before 1.2 Ma, followed by a mixing of 23- and 41-kyr cycles during the mid-Pleistocene. After 0.9 Ma, the 100-kyr glacial–interglacial cycles became dominant relative to the already present 41- and 23-kyr periodicities. The durations and rhythms of the interglacial climate varied significantly across the MPT. The past eight interglacials (MIS 21–1) are characterized by reduced precession-band variance and long durations (30–60 kyr) compared to precession-dominated interglacials before the MPT. Fig. 6 Variations of proxy data and model results over the past 1.7 Ma. a Summer insolation at 65°N [55] . b Simulated mean annual precipitation (MAP) and c mean annual temperature (MAT) over the northern China. d JY loess δ 13 C IC record. e Benthic δ 18 O stack [3] . The gray bar denotes the mid-Pleistocene transition Full size image The timing and duration of the MPT is well illustrated using continuous wavelet transforms (Methods and Fig. 7 ). Unlike the classical expression of a shift from 41- to 100-kyr cycles revealed by the benthic δ 18 O stack, our loess δ 13 C IC records document a diverse shift of the dominant periodicity from 23- to 100-kyr cycles across the MPT. In the loess δ 13 C IC spectrum, the 23-kyr cycles were dominant before 1.2 Ma and weakened after 0.7 Ma, in contrast to the persistent precession cycles in the summer insolation spectrum. Meanwhile, the 100-kyr power initiated at 1.2 Ma and became dominant after 0.7 Ma. The benthic δ 18 O spectrum, however, shows that the dominant periodicity shifted from 41-kyr cycles before 1.2 Ma to 100-kyr cycles after 0.7 Ma. While the timing and duration of the MPT are similar between terrestrial and marine records, different transitions in the frequency domain point to unique mechanisms governing the East Asian monsoon–vegetation responses to astronomical and coupled ice/CO 2 forcing. Fig. 7 Wavelet power spectra. a Summer insolation [55] , b simulated MAP, c simulated mean annual temperature, d loess δ 13 C IC , and e benthic δ 18 O stack [3] Full size image Astronomical parameters and lower boundary configurations are key factors affecting orbital-scale monsoon variability [16] , [17] , [18] , [19] . To test the plausible links of the monsoon–vegetation variability to changing insolation and ice sheets, we performed cross-wavelet analyses of the loess δ 13 C IC with summer insolation and the benthic δ 18 O. Cross-wavelet spectra reveal that over the Pleistocene the 23- and 41-kyr cycles in the δ 13 C IC records show strong coherence with the precession and obliquity signals, while remarkable glacial–interglacial fluctuations at both the 100- and 41-kyr periodicities started to be highly coupled with the benthic δ 18 O stack after the MPT (Fig. 8 ). Different coherency of the loess δ 13 C IC with summer insolation and the benthic δ 18 O mainly in the 100-kyr band suggests that evolving glacial boundary conditions across the MPT may have diminished the climate sensitivity to astronomical forcing by placing strong ice/CO 2 constraints on the coupled monsoon–vegetation system. Fig. 8 Cross wavelet spectra. a JY loess δ 13 C IC vs. summer insolation [55] , b JY loess δ 13 C IC vs. benthic δ 18 O stack [3] . Black contours indicate the coherence above 5% significance level Full size image The major differences of these forcing factors across the MPT are the ice extent and CO 2 concentration during glacial maxima [3] , [58] . Thus sensitivity analyses were based on full glacial–interglacial ranges of the ice levels (1–11) and CO 2 concentrations (180–280 ppmv) after the MPT and half ranges of the ice levels (1–6) and CO 2 concentrations (220–280 ppmv) before the MPT. Sensitivity results indicate that the MAT is primarily determined by both precession and CO 2 , and to a lesser extent by ice, and the MAP is mainly driven by precession and less by ice and CO 2 (Fig. 9 ). The coupled ice/CO 2 impact on the MAT is largely attributed to the CO 2 change, whereas their impact on the MAP is a combination of both ice and CO 2 changes. Most remarkable differences across the MPT are the decreased sensitivities of both the MAP and MAT to precession forcing and the increased sensitivities of only the MAT to the CO 2 and coupled ice/CO 2 forcing. MAT is thus less sensitive to precession forcing after the MPT when the Northern Hemisphere was more glaciated. Fig. 9 Sensitivity of temperature and precipitation to astronomical, ice, and CO 2 forcing. 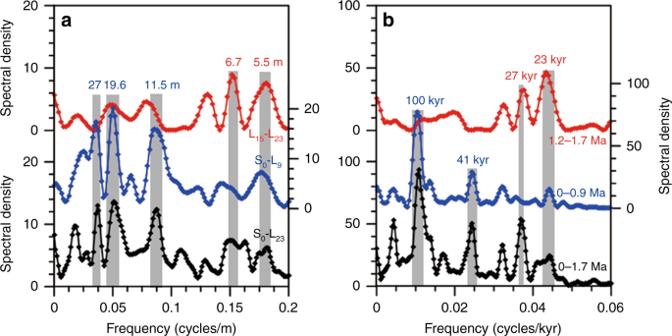Fig. 4 Spectral results of JY δ13CICrecord.aOn depth scale, dominant cyclicity changes from 5.5 to 6.7 m/cycle below L15to 19.6-27 m/cycle above L9.bThe dominant cyclicity on age scale is evidently shifted from 23-kyr before 1.2 Ma (below L15) to 100-kyr after 0.9 Ma (above L9) a Mean annual temperature (MAT) and b mean annual precipitation (MAP) responses to precession and obliquity, ice, CO 2 , and coupled ice/CO 2 forcing. Temperature and precipitation variances are spited into contributions for precession, obliquity, ice, CO 2 , and coupled ice and CO 2 variation before the MPT (pre-MPT, gray) and after the MPT (post-MPT, blue), respectively. The combined ice/CO 2 contribution is not estimated by simply adding up the individual impacts of ice and CO 2 because their effects can partly cancel out each other Full size image Different sensitivities of the MAP and MAT changes to precession, ice, and CO 2 forcing can lead to diverse manifestations in the amplitude and frequency domains across the MPT (Fig. 6 ). The simulated MAP over northern China during the last 1.7 Ma shows a persistent 23-kyr periodicity, while the ice/CO 2 modulation on the MAP became distinctive during glacial periods after 0.9 Ma. By contrast, the simulated MAT change exhibits relatively warm interglacials during 1.5–0.9 Ma and an increase in glacial–interglacial amplitude after the mid-Brunhes event (~0.42 Ma) [59] . Wavelet spectra of the simulated MAP and MAT reveal a distinctive transition from a dominant 23-kyr periodicity before 1.2 Ma to combined 23- and 100-kyr cycles after 0.7 Ma (Fig. 7 ). Filtered 100- and 23-kyr components in these proxies confirm that the onset of the 100-kyr cycle across the MPT is evident in the loess δ 13 C IC , and simulated MAT and MAP, while the 23-kyr cycle is less evident in the benthic δ 18 O than other three proxies (Supplementary Fig. 10 ). As the MAT and MAP are two important factors affecting the vegetation growth over the CLP, their frequency changes are imprinted in the δ 13 C IC record as a transition from the dominant 23-kyr to combined 23-, 41-, and 100-kyr cycles across the mid-Pleistocene. In summary, our loess δ 13 C IC time series, for the first time, illustrate a transition of coupled monsoon–vegetation changes from a dominant 23-kyr periodicity to the combined 23-, 41-, and 100-kyr cycles during the mid-Pleistocene, differing from the well-known MPT from 41- to 100-kyr cycles in most marine-based proxy records. While the MPT was usually associated with an increase in ice volume denoted by addition of 41- and 100-kyr variances in the benthic δ 18 O record, sensitivity experiments indicate that the ice impacts on the MAT and MAP over northern China did not vary significantly across the MPT. Rather, the large-amplitude 100-kyr cycle in loess δ 13 C IC is likely attributed to the amplified effect of glacial–interglacial CO 2 changes on the MAT. Proxy-model comparison reveals that the monsoon–vegetation changes responded dominantly to astronomical forcing before the MPT when the ice and CO 2 variability was relatively small. After the MPT, however, the precession forcing was attenuated by the coupled ice–CO 2 effects. Our results highlight varied roles of insolation and coupled ice/CO 2 factors in driving the temperature and hydroclimate changes from the natural past to the anthropogenic future. Drilling and sampling In 2008, we drilled a 430-m core with a recovery rate of 98% at the highest tableland near Jingyuan County. The core consists of a 427-m loess deposits underlain by 3-m gravel layer. Since the recovery rate for the upper 40-m is <85%, we investigated a nearby 40-m outcrop to collect powder samples spanning the last interglacial–glacial cycle. Continuous U-channel samples were taken from the split core sections (40–427 m) for alternating-field magnetization (AFD) measurement. Discrete samples were also collected at 0.5-m intervals using nonmagnetic quartz tubes for thermal demagnetization (THD) measurement. An upcore orientation mark was scribed on the U-channel and tube samples to provide a vertical reference. Magnetic measurements Using a MFK1-FA Kappabridge equipped with a CS-3 high-temperature furnace, temperature-dependent susceptibility ( κ – T ) curves were measured in an argon atmosphere from room temperature up to 700 °C with a heating rate of 11 o C/min and then back to room temperature. Hysteresis loops and the first-order reversal curve diagrams were obtained using a MicroMag 3900 automated vibrating sample magnetometer in a maximum field of 1000 mT. Stepwise isothermal remanent magnetization acquisition and direct current demagnetization of saturation isothermal remanence was conducted on the same samples. Hysteresis parameters were calculated after subtracting paramagnetic contributions. A Day plot was used to estimate the domain state and grain size of the magnetic particles. Stepwise thermal demagnetization was performed on the tube samples from room temperature up to 620–640 °C using a Thermal Demagnetizer (ASC TD-48). The U-channel samples were subjected to progressive AFD at peak fields up to 90 at 2.5–10-mT intervals. The natural remanence of the tube and U-channel samples was measured using a 2 G Enterprises Model 755 cryogenic magnetometer in a magnetically shielded room (<150 nT). 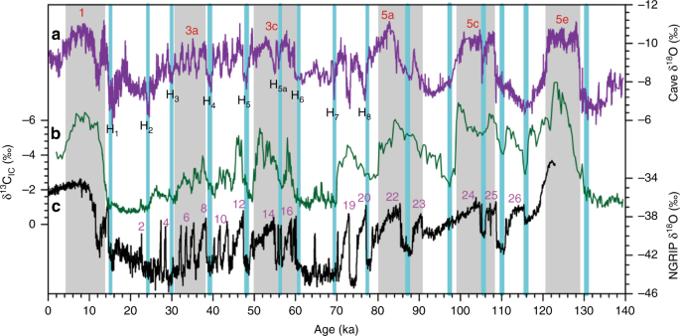Fig. 5 Proxy variations over the last 140 ka from Greenland ice core, Chinese loess, and speleothem.aChinese spleothem δ18O record15.bJY loess δ13CIC.cGreenland ice-core δ18O record53. Dashed lines denote correlations of positive loess δ13CICand speleothem δ18O with low Greenland temperature Most samples exhibit a weak viscous overprint, which can be removed at the alternating field of 20 mT or at thermal treatment with temperature >300 °C. Principal component analysis, calculated with a least square linear fit, was performed on the demagnetization data. The characteristic remanent magnetization directions were determined by a least-square fitting of the THD results between 300 and 585 °C and of the AFD between 20 and 90 mT, with a maximum angular deviation <15°. 26 Al/ 10 Be burial dating Several kilograms of quartz-bearing sediments were collected from the gravel layer underlying the Jingyuan loess sequence. The quartzose sand and gravel samples were selected for crushing and then the 0.25–0.50-mm fractions were isolated for further purification. Carbonates were dissolved with HCl and magnetic minerals were removed using magnetic separation. The quartz fractions were then leached repeatedly in hot agitated 5% HF/HNO 3 overnight. The purified quartz fraction was dissolved in 5:1 HF/HNO 3 and spiked with ~0.3 mg 9 Be. An aliquot was taken for determining the aluminum content using inductively coupled plasma–atomic emission spectrometry. After evaporation and fuming of the remaining solution in HClO 4 , Al and Be were separated on ion-exchange columns in 0.4 M oxalic acid, precipitated as hydroxides, and transformed to oxides in a furnace at 900 °C. BeO was mixed with niobium and Al 2 O 3 with copper powder for 10 Be/ 9 Be and 26 Al/ 27 Al measurement by accelerator mass spectrometer at Xi’an AMS Center, Institute of Earth Environment, Chinese Academy of Sciences. An alternative age model A different age model applied to the JY loess–paleosol sequence would generate a shift similar to the classic MPT from 41-kyr to 100-kyr cycles. In this case, the duration of the lower portion (below L 15 ) needs be extended from 480 kyr (AGE1, 1.25–1.73 Ma) to 950 kyr (AGE2, 1.25-2.2 Ma) (Supplementary Fig. 5 ). On the AGE1 model, the lower portion of the JY loess core is correlated to L 15 –S 23 , whereas on the AGE2 model, this portion is correlated to L 15 –S 29 . We prefer the first age model (AGE1) because of two reasons. First, the Olduvai subchron is not recorded in the Jingyuan loess sequence and thus the basal age should be <1.77 Ma. Second, a remarkable shift of the sedimentation rate from 13.5 to 25 cm/kyr around L 15 based on the JY-AGE2 is significantly different from the relative stable sedimentation rates in several classic loess profiles since the Olduvai subchron (Supplementary Fig. 6 ). Such a two-fold increase of the sedimentation rate at this single site cannot be explained by either tectonic or climatic factors. In addition, numerous geomorphologic and paleomagnetic investigations on the terrace sequences of the Yellow River indicate that the loess sequences (S 0 –S 24 ) accumulated on the oldest terrace are <1.8 Ma [28] , [41] Based on the new terrace classification of the Yellow River [41] , Jingyuan loess sequences (S 0 –S 23 ) was accumulated on the ninth terrace, with a rough basal age of 1.7 Ma. While an alternative pedostratigraphic correlation of the lower portion below L 15 can generate a classical MPT shift from 41-kyr to 100-kyr cycles, the relatively old basal age (~2.2 Ma) and two-fold increase in the sedimentation rates around L 15 are apparently inconsistent with independent dating results and with age–depth relationships of other classic loess profiles on the CLP, respectively. Thus we think that our preferred AGE1 is more reasonable, as inferred from the paleomagnetic and burial dating results. Spectral and wavelet analyses Spectral analysis was conducted using the Redfit 3.5 software [60] . Wavelet analyses of loess δ 13 C IC , simulated MAT and MAT, benthic δ 18 O [3] , and summer insolation [55] were performed using MATLAB codes [61] and a Morlet software package [62] . In order to visualize amplitude and frequency modulations, these data sets, except for the summer insolation, were preprocessed to isolate the 100-, 41-, and 21-kyr components using band-passing filters with central frequencies of 0.001, 0.025, and 0.05/kyr and bandwidths of 0.0002, 0.005, and 0.01/kyr before performing the wavelet transforms. The filtered signals are concentrated at three primary astronomical bands and then summed up for wavelet transforms. This preprocessing procedure can reduce the contribution of non-astronomical frequencies in the input signals and therefore improve the calculated power of three astronomical components in the paleoclimatic time series. Wavelet transform coherence was analyzed to assess high-amplitude responses of the loess δ 13 C IC , benthic δ 18 O and summer insolation at three orbital bands. Sensitivity experiments We use 61 sensitivity experiments designed to sample efficiently changes in the astronomical configurations, CO 2 concentrations, and Northern Hemisphere glaciations experienced during the Pleistocene [54] (Supplementary Fig. 8 ). Each experiment is 300-year long and we retained averages over the last 100 years for subsequent analysis. The level of Northern Hemisphere glaciations is represented by one variable called “glaciation index,” and which refers to the 1 of the 11 stages of increasing glaciation sampled from the past glacial–interglacial cycle [63] . Level 1 is the Holocene, and level 11 is the Last Glacial Maximum. We note that the configuration choice is such that ice extent grows mainly between stages 1 and 3, while ice thickness growth mainly between levels 3 and 11. Hence, by applying this design to represent ice volume changes during the early Pleistocene, we formulate the hypothesis that area fluctuations of ice sheets before the MPT were similar to after the MPT, but their thickness was smaller. The sensitivity of the monsoon climate to the full spectrum of climatic conditions experienced during the Pleistocene is estimated using the climate model HadCM3 [64] . The atmospheric component dynamics are resolved on a 3.75° × 2.5° longitude–latitude grid, and the oceanic component has a horizontal resolution of 1.25° × 1.25°. The HadCM3 has been shown to capture well enough the monsoon–ENSO interaction [65] and natural variability of the summer rainfall over China [66] . Compared to observations, the summer subtropical anticyclone in HadCM3 is too strong as in many other models. This circulation anomaly tends to induce much rainfall over the maritime continent, but the error in North China turns out to be very small (<1 mm/day) and thus quite acceptable for our purpose. In order to generate a forcing-response scenario over the Pleistocene, we scaled the benthic δ 18 O stack [3] to estimate the glaciation index over the last 1.7 Myr. CO 2 concentration over the past 0.8 Ma is obtained from Antarctic records [56] , [57] . The CO 2 before the 0.8 Ma was extrapolated to follow a linear relationship between ice volume and CO 2 concentrations over the past eight glacial cycles (Supplementary Fig. 8 ). The MAP and MAT values are the estimated equilibrium responses of HadCM3 for forcing conditions spanning the last 1.7 Ma by steps of 1 kyr. Validation for the MAT and MAP over northern China suggests that temperature is overall easier to predict than precipitation changes (Supplementary Fig. 9 ). 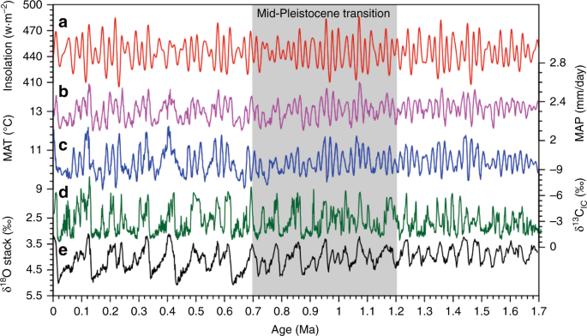Fig. 6 Variations of proxy data and model results over the past 1.7 Ma.aSummer insolation at 65°N55.bSimulated mean annual precipitation (MAP) andcmean annual temperature (MAT) over the northern China.dJY loess δ13CICrecord.eBenthic δ18O stack3. The gray bar denotes the mid-Pleistocene transition Indeed, the annual precipitation response results from partly compensating trends in winter and summer. 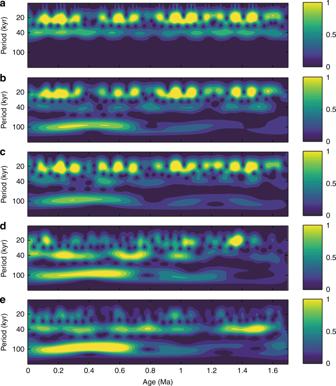Fig. 7 Wavelet power spectra.aSummer insolation55,bsimulated MAP,csimulated mean annual temperature,dloess δ13CIC, andebenthic δ18O stack3 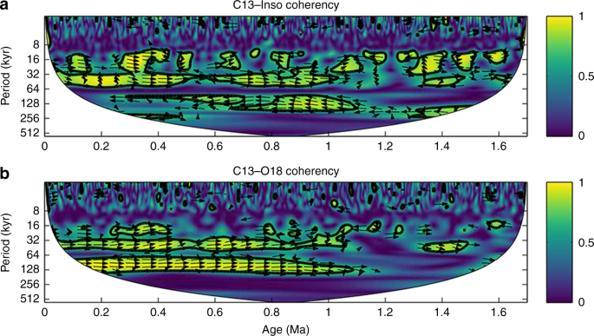Fig. 8 Cross wavelet spectra.aJY loess δ13CICvs. summer insolation55,bJY loess δ13CICvs. benthic δ18O stack3. Black contours indicate the coherence above 5% significance level 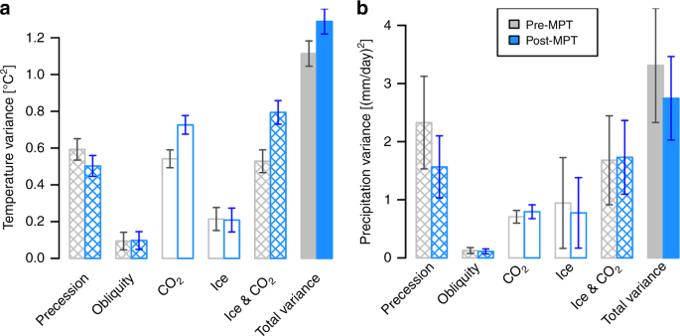Fig. 9 Sensitivity of temperature and precipitation to astronomical, ice, and CO2forcing.aMean annual temperature (MAT) andbmean annual precipitation (MAP) responses to precession and obliquity, ice, CO2, and coupled ice/CO2forcing. Temperature and precipitation variances are spited into contributions for precession, obliquity, ice, CO2, and coupled ice and CO2variation before the MPT (pre-MPT, gray) and after the MPT (post-MPT, blue), respectively. The combined ice/CO2contribution is not estimated by simply adding up the individual impacts of ice and CO2because their effects can partly cancel out each other Annual changes are therefore smaller than seasonal changes and more difficult to detect over the internal model variability background. Error bars on the variances of the MAT and MAP correspond to the error variance of the emulator estimates. They combine internal model variability, which affects the values of the 100-year long averages used to calibrate the emulator. Uncertainty might come from the fact that we only have a limited number of experiments to map the sensitivity of HadCM3 to continuous changes in input variables.